A palette of fluorescent proteins optimized for diverse cellular environments To perform quantitative live cell imaging, investigators require fluorescent reporters that accurately report protein localization and levels, while minimally perturbing the cell. Yet, within the biochemically distinct environments of cellular organelles, popular fluorescent proteins (FPs), including EGFP, can be unreliable for quantitative imaging, resulting in the underestimation of protein levels and incorrect localization. Specifically, within the secretory pathway, significant populations of FPs misfold and fail to fluoresce due to non-native disulphide bond formation. Furthermore, transmembrane FP-fusion constructs can disrupt organelle architecture due to oligomerizing tendencies of numerous common FPs. Here, we describe a powerful set of bright and inert FPs optimized for use in multiple cellular compartments, especially oxidizing environments and biological membranes. Also, we provide new insights into the use of red FPs in the secretory pathway. Our monomeric ‘oxFPs’ finally resolve long-standing, underappreciated and important problems of cell biology and should be useful for a number of applications. Since the cloning of green fluorescent protein (GFP) [1] , fluorescent proteins (FPs) have become standard imaging tools for cell biologists. FPs have been engineered to be brighter, faster folding and to cover the range of the visible spectrum [2] , [3] , [4] , [5] . Simultaneously, advanced microscopy techniques have pushed the boundaries of scientific questions that cell imaging techniques can be used to investigate. However, the range of subcellular environments within a cell pose a unique set of challenges for exploiting the full potential of FPs. Engineered FPs have been developed in the context of the cytoplasm of bacteria. In the absence of selective pressures, it is unsurprising that many FPs are not equally adapted to all cellular compartments. Recently, we reviewed the adverse impact of the chemically and physiologically distinct subcellular environments on FPs [6] . For example, the eukaryotic secretory pathway, mitochondrial inner membrane space and periplasm of gram-negative bacteria are all oxidizing environments that promote disulphide bond formation. Endocytic and secretory compartments maintain acidic pH values well below that of the cytoplasm. Within the secretory pathway, N-glycans are appended to asparagines. Another concern for many secretory fusion proteins is that localization of FPs to a membrane increases local effective protein concentrations and enhances FP tendencies to oligomerize. To quantitatively study fusion protein levels and behaviours [7] within subcellular compartments, it is vital to use FPs that properly fold, fluoresce and do not perturb the organization of the compartments. While each cellular sub-compartment poses its own challenges for FPs, the eukaryotic secretory pathway arguably encompasses the greatest variety of challenges to FPs. Nascent secretory proteins enter the lumen of the endoplasmic reticulum (ER), where the proteins will encounter ER chaperones, which assist in protein folding, as well as the acquisition of posttranslational modifications, that is, N-linked glycosylation and disulphide bond formation. There is no general consensus sequence to identify cysteines appropriate for disulphide bond formation. As a result, a secretory pathway targeted cytoplasmic protein that contains cysteines is at risk for the formation of disulphide bonds that do not occur in the cytoplasm. Similarly, nascent proteins that contain a N-X-S/T consensus sequence, where X is any amino acid except proline, will be modified with a bulky sugar attached to the asparagine [8] . These sugars can impact protein folding, stability, function and increase protein size, leading to potential steric problems [9] , [10] . Furthermore, nascent secretory proteins traverse the organelles that compose the secretory pathway, exiting the ER and entering the Golgi complex (GC) before continuing onward to vesicles and to the cell surface. During subcellular trafficking, membrane and soluble native secretory proteins are subject to quality control and the activities of resident proteins. Therefore, our study of optimizing FPs for the eukaryotic secretory pathway allowed us to determine the consequences of (1) the oxidizing environment, (2) non-native posttranslational modifications and (3) intracellular trafficking on FP folding and behaviour. Most FPs contain at least one cysteine residue. Members of the family of Aequorea victoria GFP-derived FPs contain two highly conserved cysteine residues (C48, C70; here and below the numbering of amino acid residues follows that of GFP) located between the end of β-strand 3 and the end of the internal chromophore-containing α-helix, respectively. In a correctly folded FP of the GFP-like family of proteins, the internal helix is encased by an 11-β stranded barrel and the cysteine residue side chains face inward [11] , [12] . A FP’s β-barrel must properly fold to produce the local environment required for the autocatalytic chromophore formation reaction to proceed and produce fluorescence [11] . Structurally, if either cysteine residue incorporates into a disulphide bond in the ER, it is highly unlikely the FP could achieve the required chromophore-forming structure. Therefore, when using FPs within the secretory pathway, it is preferable to select FPs that naturally lack cysteine residues, such as the family of mFruit FPs [13] or are resistant to disulphide bond formation, such as superfolder GFP (sfGFP) [14] , [15] . An alternative approach has been to engineer cysteine-less FP variants [16] , [17] . However, these efforts are complicated by the observation that, despite no obvious structural role for the cysteines, mutation of cysteines to most other amino acids decreases FP fluorescence brightness or a dark protein [18] . The currently available disulphide-resistant FP options do not cover many wavelengths and tend to be relatively dim. The mFruit FPs are relatively bright, but have been observed in aggregate-like structures [6] , [19] , [20] . As a consequence, mCherry and other mFruits have been thought to disrupt secretory pathway organelle structures [6] . We revisit these observations and reinterpret this phenomenon in this study. More commonly, many FPs are prone to non-covalent dimerization. To engineer monomeric FPs, many FPs have been extensively mutated to disrupt native dimeric and tetrameric tendencies. In GFP-derived FPs, the A206K mutation robustly prevents dimerization at the hydrophobic interface of the β-barrel [21] . Popular red FPs (RFPs), including DsRed, TagRFP, and tdTomato [13] , [22] , [23] were originally isolated as dimeric or tetrameric proteins from Anthozoa corals. Efforts by several research groups have sought to engineer more monomeric RFPs by disrupting the dimerizing protein interfaces [13] , [24] . We, and others, have examined the monomeric characteristics of FPs in live cells and have identified circumstances where previously characterized monomeric FPs are prone to non-covalent interactions [23] , [25] , [26] , [27] . Furthermore, some RFPs, like mNeptune, develop significant pools of dead-end products of chromophore formation that happen to fluoresce green [28] , a highly undesirable characteristic for imaging multiple FPs. Unfortunately, many popular FPs contain features that we hypothesized would be suboptimal for use in the distinct chemical environments of cellular organelles. In particular, many FPs contain cysteines and consensus N-linked glycosylation sequences and these may adversely impact FPs and associated reporters. In this study, we investigated these issues and sought to identify several FP colour variants for use in a variety of cellular environments. To identify suitable FPs for multiple colour labelling strategies to compliment sfGFP, we turned our attention to blue FPs (BFPs). In this study, we have engineered and improved blue (EBFP2), cyan (Cerulean), yellow (Venus) and green (sfGFP) [14] , [29] , [30] , [31] for diverse cellular environments to create a toolbox of inert FPs suitable for quantitative imaging of fluorescent fusion proteins in live cells. ER-localized FPs form inappropriate disulphide bonds Our overarching goal was to identify or develop a palette of FPs suitable for multicolour imaging of fusion proteins in the secretory pathway. Previously, we established that the cysteines in sfGFP are resistant to disulphide bond formation in oxidizing environments [15] . To test additional colours of FPs, we began with the blue FP, EBFP2 (ref. 29 ). It also contains the superfolder mutations. Therefore, we hypothesized it would also be resistant to disulphide bond formation. We directed EBFP2 to the ER of the mammalian secretory pathway with the prolactin signal sequence fused upstream of the FP and a robust ER-retrieval motif (amino-acid residues, -KDEL), to the extreme carboxy (C) terminus ( Fig. 1a ). When ER–EBFP2 was expressed in U-2 OS cells, we observed fluorescence in a typical ER tubular network distribution ( Fig. 1b ). Similar results were observed for ER–Cerulean and ER–Venus ( Supplementary Fig. 1a ). However, an immunoblot revealed a significant portion of EBFP2, under nonreducing conditions, migrated as multiple higher molecular weight species, in contrast to an expected single monomeric size ( Fig. 1c , oligomers). Nonreducing immunoblot results of lysates of cells expressing ER–mGFP, –Cerulean and –Venus also produced higher molecular weight bands ( Supplementary Fig. 1b ). The molecular weights observed suggest the formation of covalent oligomers corresponding to FP dimers, trimers and higher oligomers. Immunoprecipitation confirmed that the higher molecular weight species were composed of interchain disulphide-bonded FP homo-oligomers ( Supplementary Fig. 2a , lane 2). Thus, the cysteines that many commonly used GFP-derived FPs contain are susceptible to form non-native covalent oligomers within the secretory pathway ( Supplementary Fig. 1c ). On the basis of previously published structural data [11] , [12] , we hypothesize that the interchain disulphide-bonded FPs are unable to properly fold and consequently remain non-fluorescent. The pool of disulphide-bonded FPs does not change to an appreciable degree over time ( Supplementary Fig. 2b ), which suggests that these species are terminal products. More importantly, superfolder mutations are not sufficient insurance against disulphide bond formation by some GFP family members. 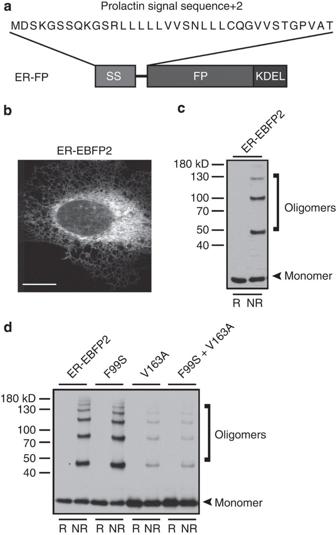Figure 1: ER-localized EBFP2 forms non-native disulphide bonds. (a) Schematic of ER-localization FP (ER–FP), containing prolactin signal sequence (SS) and KDEL retrieval motif. (b) Representative image of transiently transfected U-2 OS cells expressing ER–EBFP2; scale bar, 10 μm. (c) Immunoblot with reducing (R, +DTT) and nonreducing (NR, −DTT) conditions illustrate the tendency of ER–EBFP2 to oligomerize under NR conditions. The lower molecular weight band denotes expected molecular weight of monomeric EBFP2 (∼25 kD). (d) Superfolder and cycle-3 mutations do not protect EBFP2 cysteine residues from inappropriate disulphide bond formation. Immunoblot of ER–EBFP2, with superfolder mutations (S30R, Y39N, N105T, Y145F, I171V) and FP versions including cycle-3 GFP mutations (F99S, V163A) forms higher molecular weight oligomers under NR conditions. Figure 1: ER-localized EBFP2 forms non-native disulphide bonds. ( a ) Schematic of ER-localization FP (ER–FP), containing prolactin signal sequence (SS) and KDEL retrieval motif. ( b ) Representative image of transiently transfected U-2 OS cells expressing ER–EBFP2; scale bar, 10 μm. ( c ) Immunoblot with reducing (R, +DTT) and nonreducing (NR, −DTT) conditions illustrate the tendency of ER–EBFP2 to oligomerize under NR conditions. The lower molecular weight band denotes expected molecular weight of monomeric EBFP2 ( ∼ 25 kD). ( d ) Superfolder and cycle-3 mutations do not protect EBFP2 cysteine residues from inappropriate disulphide bond formation. Immunoblot of ER–EBFP2, with superfolder mutations (S30R, Y39N, N105T, Y145F, I171V) and FP versions including cycle-3 GFP mutations (F99S, V163A) forms higher molecular weight oligomers under NR conditions. Full size image Optimization of EBFP2 for oxidizing environments EBFP2 was previously evolved from EBFP [32] and contains the sfGFP mutations (S30R, Y39N, N105T, Y145F, I171V and A206V), plus eight additional amino-acid substitutions for a total of 14 amino-acid residue changes distinct from EGFP [33] . We sought to engineer an inert EBFP2 suitable for the ER environment and further compared EBFP2 and sfGFP for differences that might account for resistance or susceptibility to disulphide bond formation. Sequence alignment analyses ( Supplementary Fig. 1c ) revealed that two common GFP mutations (F99S and V163A) were absent from EBFP2. These missing mutations that are included in the GFP variant termed ‘cycle-3’ GFP (or αGFP [34] ) were identified using a DNA shuffling technique to introduce amino-acid mutations, F99S, M153T and V163A [35] . Crameri et al. [35] originally proposed that the three amino-acid substitution combination reduced aggregation and therefore increased chromophore maturation. We incorporated the missing two mutations and evaluated the susceptibility of forming covalent oligomers when localized to the ER. We found that these mutations did not prevent oligomer formation ( Fig. 1d ), but we observed a significant reduction in the proportion of covalent oligomers compared with monomeric species. Therefore, it appeared that we would need to mutate the two FP cysteine residues (C48 and 70). However, mutagenesis of the cysteines in the closely related EGFP decreased brightness with single cysteine mutations and rendered the protein dark upon mutating both cysteines [18] . Similarly, when we mutated cysteines in mTagBFP into secBFP2 (ref. 17 ), the resulting brightness was greatly diminished relative to parental mTagBFP, which was engineered from TagRFP [36] . Indeed, cysteine to serine substitutions diminished the fluorescent signal of the cysteine-less EBFP2 ( Table 1 ). Reverse mutagenesis revealed that C70 was sensitive to mutagenesis and responsible for the decreased fluorescence. Cysteine is often more hydrophobic than what its structure intuitively suggests [37] . Thus, we considered more hydrophobic mutations. A valine mutation was better tolerated than the amino-acid substitutions of serine or alanine. When expressed in the cytoplasm of cells, the C48S/C70V variant had lower relative brightness compared with the parental cysteine-containing EBFP2. In an attempt to restore fluorescence, we turned our attention to the missing F99S and V163A cycle-3 mutations. Additional rounds of mutagenesis revealed that the combination of C48S, C70S and V163A resulted in a BFP with brightness comparable to parental EBFP2, without the problematic cysteine residues ( Table 1 ). Table 1 Overview of EBFP2 mutants and fluorescence intensities. Full size table Importantly, the new BFP, termed oxBFP, is fluorescent within the cytoplasm and lumen of the ER and does not participate in non-native disulphide bonds ( Fig. 2a,b ). Spectral characterization of oxBFP was conducted to confirm that the spectral properties remained unchanged compared with the parental EBFP2. We observed a modest decrease in photostability under comparable imaging parameters ( Fig. 2c ). OxBFP maintained the absorbance ( Fig. 2d ), excitation and emission ( Fig. 2e ) spectra of EBFP2, confirming the incorporated mutations did not affect the spectral properties of the FP. 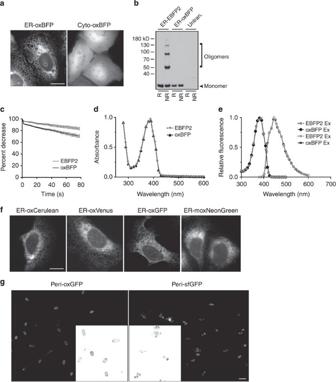Figure 2: OxFPs are fluorescent. (a) Representative image of ER–oxBFP and Cyto-oxBFP expressing U-2 OS cell; scale bar, 10 μm. (b) Immunoblot of cells transfected with ER–EBFP2 or –oxBFP. Under nonreducing conditions, the optimized, cysteine-less oxBPF does not form inappropriate disulphide bonds; untran., untransfected. (c) oxBFP (black line) maintains moderately comparable photostability properties under standard imaging conditions compared with EBFP2 (grey line). Optimized oxBFP variant (black data points) has comparable spectral characteristics to parental EBFP2 variant (grey data points). (d) Absorbance measurements and (e) fluorescence excitation (closed data points) and emission (open data points). (f) Representative images of ER–oxCerulean, –oxVenus, –oxGFP or moxNeonGreen expressing U-2 OS cells. Scale bar, 10 μm. (g) oxGFP fluoresces homogenously throughout the periplasm of gram-negative bacteria (CodonPlus competent, BL21 RP). Cells were induced for 1 h with IPTG and then imaged. Inset thumbnails are enlarged and inverted for detail. Scale bar, 1 μm. Figure 2: OxFPs are fluorescent. ( a ) Representative image of ER–oxBFP and Cyto-oxBFP expressing U-2 OS cell; scale bar, 10 μm. ( b ) Immunoblot of cells transfected with ER–EBFP2 or –oxBFP. Under nonreducing conditions, the optimized, cysteine-less oxBPF does not form inappropriate disulphide bonds; untran., untransfected. ( c ) oxBFP (black line) maintains moderately comparable photostability properties under standard imaging conditions compared with EBFP2 (grey line). Optimized oxBFP variant (black data points) has comparable spectral characteristics to parental EBFP2 variant (grey data points). ( d ) Absorbance measurements and ( e ) fluorescence excitation (closed data points) and emission (open data points). ( f ) Representative images of ER–oxCerulean, –oxVenus, –oxGFP or moxNeonGreen expressing U-2 OS cells. Scale bar, 10 μm. ( g ) oxGFP fluoresces homogenously throughout the periplasm of gram-negative bacteria (CodonPlus competent, BL21 RP). Cells were induced for 1 h with IPTG and then imaged. Inset thumbnails are enlarged and inverted for detail. Scale bar, 1 μm. Full size image A palette of oxidizing environment-optimized FPs To expand the available FP colours for oxidizing environments, we applied the same approach to Cerulean and Venus FPs by synthesizing versions that were human codon optimized and contained the sfGFP and cysteine to serine mutations to create oxCerulean and oxVenus. We also removed the cysteines from sfGFP to create, oxGFP. Although, our previous results established that the cysteines in the sfGFP were protected, we sought to create a GFP insusceptible to disulphide bond formation. In addition, we were able to create a cysteine-less green alternative to GFP family members, moxNeonGreen, an oxidizing environment-optimized variant of the recently described mNeonGreen [38] . We successfully expressed and localized the new FPs to the ER ( Fig. 2f ) and determined that the spectral characteristics of the cysteine-less FPs were comparable to the parental FPs ( Supplementary Fig. 3 ). Table 2 summarizes the spectral properties of the new palette of oxidizing-optimized oxFPs: blue oxBFP, green oxGFP, green moxNeonGreen, cyan oxCerulean and yellow oxVenus. Table 2 Properties of oxidation-resistant fluorescent proteins. Full size table In addition to the ER, other cellular compartments can be oxidizing, including the periplasm of gram-negative bacteria. We previously found that sfGFP fluoresces robustly in the periplasm of gram-negative bacteria [15] . We tested the utility of oxGFP in the periplasm of bacteria and we found that oxGFP fluoresces equally well ( Fig. 2g ). We predict that the other oxFP variants should also be useful for studies in the bacterial periplasm. Consequences of disulphide bond formation The higher molecular weight bands observed by immunoblots ( Figs 1 and 2 , Supplementary Fig. 1 ) established that significant fractions of non-optimized FPs misfold in oxidizing compartments. Comparisons of fluorescence intensity measurements revealed a decrease of fluorescence signal in cells transiently expressing the non-optimized FP variant. Cells expressing ER–EBFP2, the non-optimized FP, are visibly dimmer compared with ER–oxBFP ( Fig. 3a,b ). Evaluation of the relative fluorescence intensity of the optimized oxBFP with EBFP2 revealed a 27% reduction in the detectable fluorescence when EBFP2 was localized to the ER compared with ER–oxBFP ( Fig. 3c ). This measurable decrease in fluorescence signal was specifically a consequence of the oxidizing environment of the ER. When the two BFPs were localized to the cytoplasm, in the absence of disulphide formation, the BFPs exhibited nearly identical mean fluorescence intensities ( Fig. 3c , inset). 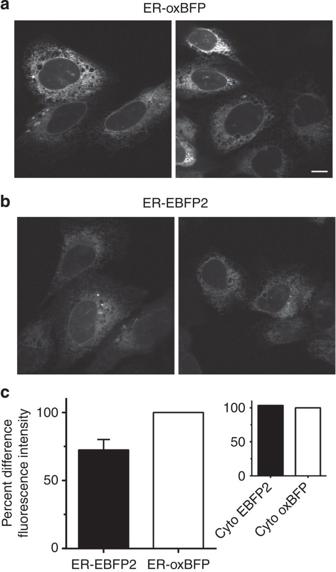Figure 3: ER-localized oxBFP has greater fluorescence intensity. Representative images taken with identical imaging conditions of live U-2 OS cells transiently transfected (16 h post transfection) with (a) ER–oxBFP or (b) ER–EBFP2 illustrate the higher fluorescence level of the cysteine-less variant; scale bar, 10 μm. (c) Quantification of the percent difference of relative mean fluorescent intensity of the ER fluorescence signal ER–EBFP2 has an∼27% decrease in brightness, totaln=250 cells (ER–EBFP2 73 cells, ER–oxBFP 72 cells, Cyto-EBFP2 43 cells and Cyto-oxBFP 62 cells). Error bars signify s.e.m. for data collected from three experimental replicates. Figure 3: ER-localized oxBFP has greater fluorescence intensity. Representative images taken with identical imaging conditions of live U-2 OS cells transiently transfected (16 h post transfection) with ( a ) ER–oxBFP or ( b ) ER–EBFP2 illustrate the higher fluorescence level of the cysteine-less variant; scale bar, 10 μm. ( c ) Quantification of the percent difference of relative mean fluorescent intensity of the ER fluorescence signal ER–EBFP2 has an ∼ 27% decrease in brightness, total n =250 cells (ER–EBFP2 73 cells, ER–oxBFP 72 cells, Cyto-EBFP2 43 cells and Cyto-oxBFP 62 cells). Error bars signify s.e.m. for data collected from three experimental replicates. Full size image Both freely diffusing luminal and membrane-localized non-optimized FPs within the secretory pathway are prone to inappropriate disulphide bond formation. We localized an optimized and a non-optimized FP to the GC with the 1,4-galactosyltransferase, GalT, signal anchor transmembrane domain ( Fig. 4a ). The tagged proteins are oriented with the FP in the lumen of the ER and GC [39] . Nonreducing immunoblots revealed that GalT–mGFP forms covalent oligomers ( Fig. 4b ). 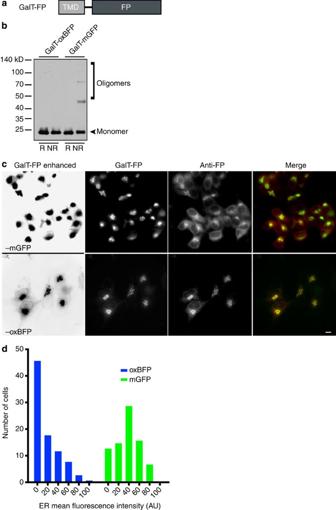Figure 4: Golgi complex membrane-localized mGFP forms inappropriate disulphide bonds and is inefficiently trafficked to the GC. (a) Schematic of GC-localized FP (GalT–FP) containing GalT transmembrane domain upstream of FP. (b) Immunoblot revealed the tendency of GalT–mGFP to form oligomers under NR conditions. Optimized, cysteine-less GalT–oxBFP does not form inappropriate disulphide bonds. (c) Representative images of HeLa cells transiently transfected with GalT–mGFP or –oxBFP. Immunofluorescence with anti-GFP revealed a significant fluorescently undetectable pool of GalT–mGFP in the ER. ER labelling by the FP is digitally enhanced with Levels tool in Photoshop in far left panels. Note that weak ER is apparent in all of the oxBFP expressing cells, but rarely observed in mGFP expressing cells. Scale bar, 10 μm. (d) Distribution of the ER fluorescence intensity values (mean fluorescence intensities of regions of anti-GFP staining proximal to the GC).n≥80 cells collected from 11 to 13 fields per construct. Figure 4: Golgi complex membrane-localized mGFP forms inappropriate disulphide bonds and is inefficiently trafficked to the GC. ( a ) Schematic of GC-localized FP (GalT–FP) containing GalT transmembrane domain upstream of FP. ( b ) Immunoblot revealed the tendency of GalT–mGFP to form oligomers under NR conditions. Optimized, cysteine-less GalT–oxBFP does not form inappropriate disulphide bonds. ( c ) Representative images of HeLa cells transiently transfected with GalT–mGFP or –oxBFP. Immunofluorescence with anti-GFP revealed a significant fluorescently undetectable pool of GalT–mGFP in the ER. ER labelling by the FP is digitally enhanced with Levels tool in Photoshop in far left panels. Note that weak ER is apparent in all of the oxBFP expressing cells, but rarely observed in mGFP expressing cells. Scale bar, 10 μm. ( d ) Distribution of the ER fluorescence intensity values (mean fluorescence intensities of regions of anti-GFP staining proximal to the GC). n ≥80 cells collected from 11 to 13 fields per construct. Full size image To investigate where the misfolded dark secretory pathway protein fusions localize, we compared where optimized and non-optimized GalT–FP reporters localize in cells. GalT–mGFP or -oxBFP exhibit predominantly compact perinuclear fluorescence, consistent with GC localization ( Fig. 4c ). Yet, immunofluorescence (IF) of the same cells with anti-GFP antibodies revealed that a substantial dark pool of GalT–mGFP resides in the ER ( Fig. 4c ) of most expressing cells ( Fig. 4d ). Although GalT–oxBFP expressing cells also exhibit some ER fluorescence by IF: (i) it is much less common, (ii) in those cells, the ER is visible in the FP channel too, especially when image levels are enhanced and (iii) each GC has a much higher mean fluorescence intensity (MFI) relative to the ER intensity. In contrast, GalT–mGFP expressing cells have comparatively higher ER fluorescence and more modest GC fluorescence by IF, with little ER fluorescence intensity visible from the FP, even when image contrast levels are enhanced. GalT–EBFP2 expressing cells also frequently exhibit an ER pool visible only in immunofluorescence images ( Supplementary Fig. 4a ). These data suggest that, in GalT–mGFP, the interchain disulphide bonds that we observed via nonreducing immunoblots ( Fig. 4b , oligomers) likely correspond to the non-fluorescent pool revealed by anti-GFP IF. Together, the representative images and quantification indicate that a substantial proportion of GalT–mGFP remains in the ER as non-fluorescent covalent oligomers, while GalT–oxBFP properly folds, fluoresces and traffics to the GC. These examples establish the importance of using the inert oxFPs for studies of secretory compartments in cells. Two-colour FP pairs for secretory protein FP fusions Commonly, dual-colour FP-fusion labelling approaches use mCherry or another RFP in combination with a GFP. MCherry does not contain cysteine residues, is reportedly monomeric [13] , and it has been successfully expressed in oxidizing environments, including bacterial periplasm [40] . Therefore, mCherry would be expected to be a suitable FP option for use in secretory protein fusions. However, for GC-localized membrane fusion proteins, we have previously found mCherry to be a potentially problematic choice, as mCherry fusions often localize to numerous punctate structures distinct from GFP family members fused to GalT [6] . Others have reported that mCherry protein fusions can aggregate [41] , impair growth in yeast and development of tissues in Xenopus laevis [27] , [42] . These issues motivated us to test the utility of our oxFPs for dual-color labelling schemes, especially for labelling the GC. For comparison, we expressed GalT–oxBFP and –mCherry fusions in HeLa cells ( Fig. 5a ). Representative images show expected ER–oxGFP labelling of the ER network along with discretely GC-localized GalT–oxBFP. In contrast, GalT–mCherry fusions localized in a dispersed pattern of puncta throughout the cell. However, at lower expression levels, especially in stably transfected cells, a mixed puncta and GC distribution can be observed for GalT–mCherry ( Supplementary Fig. 4b ). Thus, oxBFP appears to be a suitable FP for use in GC reporters. 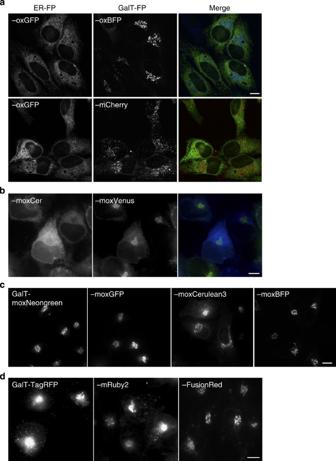Figure 5: Golgi complex-localized membrane fusions with oxBFP exhibit significant differences relative to red FP fusions. Representative image of (a) HeLa cells transiently co-expressing ER–oxGFP and GalT–oxBFP or –mCherry. (b) Live cells expressing GalT–moxVenus and ER–moxCerulean3 are readily distinguishable and thus represent a useful pair of FPs for two-colour imaging in the secretory pathway of live cells. (c) Transiently transfected HeLa cells expressing GalT–moxNeonGreen, –oxGFP, –moxCerulean3, –moxBFP. (d) Live cells expressing GalT–TagRFP or GalT–mRuby2 exhibit both the GC and bright puncta throughout the cell, while GalT–FusionRed appears to primarily localize to GC structures. Scale bar, 10 μm. Figure 5: Golgi complex-localized membrane fusions with oxBFP exhibit significant differences relative to red FP fusions. Representative image of ( a ) HeLa cells transiently co-expressing ER–oxGFP and GalT–oxBFP or –mCherry. ( b ) Live cells expressing GalT–moxVenus and ER–moxCerulean3 are readily distinguishable and thus represent a useful pair of FPs for two-colour imaging in the secretory pathway of live cells. ( c ) Transiently transfected HeLa cells expressing GalT–moxNeonGreen, –oxGFP, –moxCerulean3, –moxBFP. ( d ) Live cells expressing GalT–TagRFP or GalT–mRuby2 exhibit both the GC and bright puncta throughout the cell, while GalT–FusionRed appears to primarily localize to GC structures. Scale bar, 10 μm. Full size image The propensity of FPs to oligomerize Since mCherry is a popular FP, we sought to carefully test the possibility that GalT–mCherry might have a tendency to oligomerize and/or aggregate. If so, oligomers or aggregates could disrupt proper localization in the GC. We examined mCherry oligomerization using the live cell assay that we recently developed for assessing FP monomericity in cells. In addition, we also tested whether other FPs were sufficiently monomeric to avoid FP oligomerization artefacts [21] , [43] . We directly compared oxFPs and oxFPs modified with the A206K GFP monomerizing mutation using an abbreviated version of our CytERM assay [26] , [38] . We found that EBFP2 and mTagBFP possess strong propensities to oligomerize and form Organized Smooth Endoplasmic Reticulum (OSER) whorl structures ( Table 3 ) ( Supplementary Fig. 4c ). The A206K mutation significantly diminished FP–FP interactions and whorl formation for oxBFP. Therefore, we subsequently monomerized all of our constructs to create monomeric oxidizing environment-optimized (mox) FPs. Table 3 Propensity of BFPs to oligomerize in mammalian cells. Full size table On the basis of our results, the tendency of GFP family members to dimerize does not appear to impact GC structure. Furthermore, we rarely observed OSER structures with CytERM–mCherry or for a newer RFP, FusionRed [3] ( Supplementary Fig. 4c ). Therefore, we consider oligomerization unlikely to explain the punctate structures observed in GalT–mCherry expressing cells. Another RFP, CytERM–mRuby2 (ref. 4 ), was highly prone to OSER formation ( Supplementary Fig. 4c ). These data were quantified using the CytERM assay ( Table 3 ). We note that the reported monomericity of mRuby2 was assessed for the parent protein, mRuby, by passing a solution of purified protein over a molecular sizing column [25] , [44] . As with another RFP, TagRFP, molecular sizing columns do not appear to be a robust method for determining the propensity of FPs to oligomerize in cells [5] . Monomeric oxFP two-colour pairs for oxidizing environments Using our new moxFPs, we tested their suitability for use in GalT reporters and for dual-colour imaging pairs. GalT–moxVenus and ER–moxCer constructs localized in patterns similar to that observed with oxGFP and oxBFP ( Fig. 5b ). Thus, the ox- and monomerized ox- FPs can be exploited for at least two different two-colour pairs for multicolour imaging. In addition, when expressed stably and transiently in cells, GalT–moxBFP, moxCerulean, moxGFP and moxNeonGreen localized predominantly to compact perinuclear GC structures ( Fig. 5c , Supplementary Fig. 4b ). We asked whether RFPs could be used for GC localization reporters by fusing the GalT domain to TagRFP, mRuby2 (ref. 25 ), and FusionRed [27] . The first two red FP fusions strongly resembled the mCherry GalT distribution while FusionRed predominantly localized in a GC pattern ( Fig. 5d ). Of these red FPs, only mCherry is cysteine-free. Thus, many RFPs appear to be suboptimal for use in the secretory pathway and even mCherry appears to be problematic when used with a GC-localized membrane protein. However, given the need for red FPs in multicolour imaging, the punctate distribution of GalT–mCherry merited further investigation before rejecting use of mCherry in the secretory pathway. Importantly, upon closer examination of the GC distribution of the other GalT–moxFP fusions, we encountered a surprising result. GalT–moxCerulean and GalT–moxCerulean3 (an improved Cerulean variant) [45] also localized to both GC and punctate structures ( Fig. 5c ). As moxCerulean3 ( Table 2 and Supplementary Fig. 5 ) is closely related to other GFP family members, this result suggested a potential explanation for the punctate pattern of GalT–mCherry that we investigate in the next section. GalT–mCherry accumulates in lysosomes RFPs are essential reagents for cell biologists and they have many desirable properties, including brightness and illumination with longer less phototoxic wavelengths that are less prone to exciting autofluorescent substrates in cells. Several of the red FPs were evolved from inherently dimeric or tetrameric proteins. For fusion proteins, it is critical that the FP of choice not oligomerize. We ( Supplementary Fig. 4c ) [26] and others [46] , [47] find that not all RFPs reported as monomeric perform as monomers in cells. We observed that mCherry only weakly oligomerizes ( Supplementary Fig. 4c and Table 3 ). Against this background, we sought to understand the behaviour of GalT–mCherry. First, we tested whether the GalT–mCherry puncta are disrupted GC membranes by staining for GC and GC/intermediate compartment markers GM130 and β-COP, respectively. Both markers robustly co-localize with the compact perinuclear GC structures labelled by the GalT fusions, but neither labels the mCherry puncta throughout the cell ( Fig. 6a,b ). These results also reveal that GalT–mCherry does not necessarily disrupt the GC. We further tested this idea by co-expressing GalT–mCherry with GalT–moxGFP. Both reporters localize to GC structures and only GalT–mCherry localizes to puncta, as well ( Fig. 6c ). Therefore, the GC remains intact and GalT–mCherry does not appear to drag other GalT reporters into puncta structures. 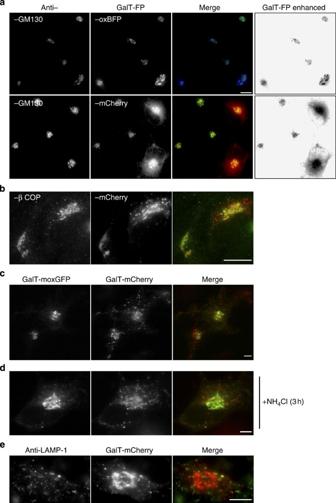Figure 6: GalT–mCherry puncta localize to lysosomes. (a) Hela cells expressing GalT–oxBFP (upper panels) or GalT–mCherry (lower panels) were fixed and stained with the GC marker anti-GM130. Co-localization was observed for GalT–oxBFP, but cells expressing moderate levels of GalT–mCherry exhibit both GC co-localization and bright puncta throughout the cell. (b) GalT–mCherry expressing HeLa cells fixed and stained for the GC and intermediate compartment marker β COP. The red puncta do not co-localize with the green β COP puncta. (c,d) HeLa cells co-expressing GalT–moxGFP and GalT–mCherry show co-localization in the GC structure, but GalT–moxGFP does not localize to red puncta. (d) Pretreatment with NH4Cl for 3 h leads to substantial co-localization of GalT–moxGFP with red puncta. (e) GalT–mcherry expressing HeLa cells were fixed and stained for the lysosomal marker anti-LAMP1. Several red puncta co-localize with the LAMP1 positive structures. Scale bar, 10 μm. Figure 6: GalT–mCherry puncta localize to lysosomes. ( a ) Hela cells expressing GalT–oxBFP (upper panels) or GalT–mCherry (lower panels) were fixed and stained with the GC marker anti-GM130. Co-localization was observed for GalT–oxBFP, but cells expressing moderate levels of GalT–mCherry exhibit both GC co-localization and bright puncta throughout the cell. ( b ) GalT–mCherry expressing HeLa cells fixed and stained for the GC and intermediate compartment marker β COP. The red puncta do not co-localize with the green β COP puncta. ( c , d ) HeLa cells co-expressing GalT–moxGFP and GalT–mCherry show co-localization in the GC structure, but GalT–moxGFP does not localize to red puncta. ( d ) Pretreatment with NH 4 Cl for 3 h leads to substantial co-localization of GalT–moxGFP with red puncta. ( e ) GalT–mcherry expressing HeLa cells were fixed and stained for the lysosomal marker anti-LAMP1. Several red puncta co-localize with the LAMP1 positive structures. Scale bar, 10 μm. Full size image Next, we revisited our data with the GalT-moxCer3 reporter, which also localized in a punctate distribution ( Fig. 5c ). Aside from spectra, a major difference between Cerulean3 (moxCer3) and other GFP family members is the exceptionally low pKa (3.2; ref. 45 ) relative to the pKa of GFPs (5.5–6). The pKa is the pH at which a fluorophore will be quenched in brightness by one half. FPs often fully quench at only slightly lower pH values. Like Cer3, mCherry has a low pKa <4.5 (ref. 13 ). In addition, mCherry is resistant to proteolysis in lysosomes, while GFP family members are highly susceptible [48] . Katayama et al. [49] reported that cytoplasmic mCherry can accumulate in lysosomes, possibly through an autophagy mechanism and that the resistance of mCherry to pH and degradation leads to an aggregate-like pattern. We considered the possibility that a similar phenomenon occurs for mCherry fused to membrane proteins in the secretory pathway. We hypothesized that GalT–FP fusions are not statically localized to the GC and could traffic to the endosomal/lysosomal system for turnover. The pH of late GC compartments and the endosomal–lysosomal system decreases from 6.5 down to 4 (ref. 50 ), which should quench the fluorescence of most GFP family members. To test whether GalT–moxGFP traffics similarly could accumulate in puncta, the pH gradient of the secretory pathway was disrupted. Treatment with NH 4 Cl for 3 h dramatically redistributed GalT–moxGFP, which now co-localized with GalT–mCherry puncta ( Fig. 6d ). Finally, we directly tested whether GalT–mCherry puncta localize in lysosomes by co-localizing with the marker anti-LAMP1 ( Fig. 6e ). Together, these observations have important implications for imaging studies in the secretory pathway. The choice of FP clearly influences the localization pattern. Our data suggest that GalT eventually traffics to the lysosome; though we cannot currently rule out the possibility that mCherry contains a cryptic lysosome-targeting sequence. GFP family members, including the new ox and mox variants, robustly label the GC with high signal/noise probably because the FPs are destroyed in lysosomes. In addition, mCherry reportedly matures more slowly than the GFP family member [51] and this property could decrease the visible pool of GalT–mCherry in the GC at a steady state. Huang et al. [52] cautioned that even the FP linker can impact FP-fusion stability and steady-state distribution. Whether the properties of a GFP family member or mCherry are advantageous or disadvantageous will depend on the goal of the experiment, though awareness of these issues will enable investigators to exploit these different properties. Therefore, when using FP fusions in experiments, it is vital to validate the behaviour of the fusion protein relative to the native protein. Finally, to confirm the utility of the moxFPs, we sought to confirm the functionality of the FPs in the cytoplasm. We found that all of the GFP family member moxFPs functioned comparably with the parental proteins when fused into standard actin and tubulin constructs and gave expected distributions of actin stress fibres and microtubules ( Supplementary Fig. 6a,b ). We had different results with mNeonGreen and moxNeonGreen. Both versions formed actin stress fibres ( Supplementary Fig. 6a ). However, neither version was significantly incorporated into microtubules ( Supplementary Fig. 7 ). In the original report [38] , it was unclear how long the linker was, but we tried both lengths and had the same result ( Supplementary Fig. 7a,b ). We recommend caution when making fusions with mNeonGreen and its variants. The new toolbox of the moxFPs, which includes moxBFP, moxCerulean3, moxVenus and moxNeonGreen, provides a powerful variety of inert options for multiple FP expression combinations for soluble and membrane FP fusions. The majority of the reported FPs contain at least one cysteine residue (with the notable exception of the DsRed/mFruit family). Despite the resulting undesirable disulphide -bonded misfolded oligomers, the higher molecular weight oligomers represent a curious protein-folding phenomenon that suggests potentially important insights into the process of FP folding in cells. A completely and correctly folded FP β-barrel structure should shield cysteines away from potential interactions. Therefore, disulphides must form between FPs before they have folded into β-barrels. The ER lumen is a highly crowded environment (100 mg ml −1 protein [53] ). As nascent FPs enter the crowded ER lumen, they will transiently contact numerous diffusing secretory proteins. We have no evidence that FPs form inappropriate disulphide bonds arbitrarily with random luminal ER proteins. We would have expected to see smears on nonreducing immunoblots, instead of discrete bands at specific molecular weights that correspond to FP interchain disulphide-bonded FP species. Disulphide-bonded FP oligomers suggest that FPs do not immediately fold into their protected native β-barrel structure. Instead, FPs likely form persistent (at least for seconds and maybe longer) one or more intermediate species (FP int ) that can oligomerize via an interface distinct from the hydrophobic dimerizing interface on the outer surface of GFP. These species are probably also recognized by resident ER chaperones. Incompletely folded GFP molecules likely interact with the complementary domains of other GFP molecules in trans . It is unclear whether the quasi-species are reversible and can eventually form two separately folded and fluorescent FPs in the cytoplasm or ER. Within the ER, cysteine residues in the FP int are exposed and could preferentially form a disulphide bond with an interacting FP int species. This scenario is especially plausible if the FP int has a high affinity for homo-oligomerization, increasing the likelihood of disulphide bonds forming between FPs, probably in cooperation with a PDI family member. To circumvent the challenges that subcellular organelles pose to FPs, we sought to optimize FP technologies. We have created a set of bright oxFPs ( Table 2 ) that can be used for quantitative multicolour labelling strategies. In the cytoplasm and non-cytoplasmic compartments, oxGFP, oxBFP, oxCerulean, moxCerulean3 and oxVenus can be reliably and robustly expressed. Furthermore, the moxFPs versions are monomeric and encode no apparent sequence-specific sites accessible for N-linked glycosylation or disulphide bond formation. The moxFPs are currently the most practical solution to reliably engineer FP fusions with soluble and membrane cellular proteins of interest. Our results emphasize the urgent need to develop better cysteine-less and robustly monomeric red FPs for use in the secretory pathway. We have extensively studied the impact of the chemically distinct and reactive environments of the eukaryotic secretory compartments on the functionality of FPs. As we explored popular FP applications, it became apparent that moxFP modifications are essential. For example, we measured a significant decrease in maximum fluorescence of non-optimized ER–EBFP2 ( Fig. 3c ). Findings with GalT–mGFP further confirm significant loss and mislocalization of functional fluorescent molecules due to the formation of non-native disulphide bonds ( Fig. 4 ). We predict that the accumulation of misfolded non-fluorescent FP molecules within the ER could lead to underappreciated off-target effects, including changes to the ER environment through titration of ER chaperones and crowding effects of aggregated misfolded proteins leading to unintended side effects on secretory resident proteins and protein trafficking. Equally importantly, the non-FP component of a dark pool of fusion proteins may remain functional and could lead to gross underestimations of the location and activity levels of fusion proteins. In such cases, the concentration of oxFP fusions expressed in cells will be most accurately defined by biochemical analysis instead of imaging analysis. For example, the observed FP-fusion fluorescence would correlate with the levels of the correctly folded monomeric species detected by immunoblot. As the optimized oxFPs do not accumulate misfolded, non-fluorescent species, total levels of fluorescence will quantitatively reflect FP-fusion levels. This last point is especially pertinent to the current thrust towards quantitative single-cell imaging for modern cell biologists. CMV promoter-driven transiently transfected plasmids have been useful for studying proteins in cells, but it remains unclear how much the behaviour of grossly overexpressed proteins accurately reflects physiologic cell and protein behaviours. New engineering technologies, especially CRISPR, have made it possible to chromosomally tag endogenous genes with FPs to enable truly physiologic expression and regulation of levels of FP-fusion proteins [54] . In the absence of CMV promoter-driven expression levels, it will be vital for each FP fusion to correctly fold and fluoresce to quantitatively visualize FP-fusions using fluorescence microscopy. Quantitative experiments to investigate cell-to-cell variation, proteomics and to help develop quantitative cellular models will require accurate censuses of cellular protein populations. FP fusions absolutely must not distort or perturb cellular compartments. The bright multicolour moxFPs developed here were motivated by these needs and represent essential tools for cell biologists studying diverse intracellular environments. Chemicals Dithiothreitol (DTT; Fisher Scientific, Pittsburgh, PA) was diluted to the indicated concentrations from a 1 M stock solution in dH 2 O. N -ethylmaleimide (NEM; Acros Organics, Thermo Fisher Scientific, Rockford, IL) was diluted to indicated concentrations from a 2 M stock in dH 2 O. Mammalian plasmids EBFP2, Cerulean, sfGFP and Venus were previously described [14] , [29] , [30] , [31] . Oxidizing-resistant FPs, EBFP2 and sfGFP, contain cysteine to serine mutations using standard site-directed mutagenesis procedures. Optimized oxCerulean, oxCerulean3, moxNeonGreen and oxVenus were synthesized by GenScript (Piscataway, NJ) and included cysteine to serine mutations, superfolder mutations, and were human codon optimized. To create cytoplasmic and ER-localized reporters, FP-encoding sequences were amplified using primers listed in Supplementary Table 1 . FP fragments were cloned into the AgeI/NotI sites of the pEGFP-N1 plasmid (Clontech, Mountain View, CA) or pER–mRFP [55] creating ER–FPs. To produce the GalT GC marker, cytoplasmic -N1 constructs were digested with SacI/AgeI and inserted into -N1 vector containing the GalT signal anchor (amino acids 1–61). FP fusions with actin or tubulin were generated from parental C1 pEGFP-actin (Clontech) and pEGFP-tubulin (Clontech) vectors. Vectors were digested with NheI/BglII. FP fragments were then cloned into NheI/BglII sites. To investigate specific amino-acid substitution consequences on FP fluorescence, reverting mutations were re-introduced into FPs using designated primers ( Supplementary Table 1 ). All the constructs were confirmed by sequencing. Bacterial cloning, expression and protein purification FP sequences were amplified using primers listed in Supplementary Table 1 . FP fragments were cloned into pEcoli-Cterm 6xHN vector (Life Technologies, Grand Island, NY) at NcoI and PstI restriction sites. Vectors were expressed in CodonPlus competent, BL21 RP host cells (Stratagene, La Jolla CA). Five-millilitre cultures were grown at 37 °C, 225 r.p.m. overnight in LB under chloramphenicol and ampicillin drug selection. One millilitre of overnight cultures was added to 50 ml of drug-free LB for 2 h at 37 °C, 225 r.p.m. For induction, 1 mM IPTG was added to the cultures and returned to 37 °C, 225 r.p.m. shaker for 4 h. Cultures were pelleted at 5,000 r.p.m. for 15 min at 4 °C. For protein purification procedure, refer to manufacturer’s protocol for His60 Ni Superflow Resin & Gravity Column manual (Life Technologies). Peri-oxGFP was generated using the same cloning strategy as previously described peri-sfGFP [15] . Cell culture and transfection U-2 OS (ATCC HTB-96), HeLa (ATCC CCL-2) and MDCK (ATCC CCL-34) cells were routinely cultured in RPMI-1640 medium (Mediatech, Manassas, VA), supplemented with 5 mM GlutaMAX (Life Technologies), penicillin/streptomycin (Invitrogen, Carlsbad, CA) and 10% heat-inactivated fetal bovine serum (Hyclone from Thermo Fisher Scientific) at 37 °C in 5% CO 2 . All the constructs were transiently transfected for 16–20 h into cells using Lipofectamine 2000 (Life Technologies) according to the manufacturer’s instructions. HeLa cells with stable expression of GalT–FPs were generated and maintained using G418 (Geneticin, Live Technologies) selection. Live cell fluorescence imaging For imaging experiments, cells were grown in eight-well LabTek coverglass chambers (Nunc, Rochester, NY). The cells were imaged in phenol red-free RPMI-1640 freshly supplemented with 10 mM Hepes (Thermo Fisher Scientific) and 10% fetal bovine serum. To increase organelle pH, when indicated, cells were incubated in media containing 20 mM NH 4 Cl and no Hepes for 3 h at 37 °C before imaging. Live cells were imaged on a 37 °C environmentally controlled chamber of a confocal microscope system (Zeiss LSM-5 LIVE microscope with Duoscan attachment; Carl Zeiss MicroImaging, Inc., Thornwood, NY) with a × 63/1.4 NA oil objective and a 405 nm 50 mW diode laser with a 415–505 nm bandpass or 510 nm longpass filter for EBFP2 and 415–475 nm bandpass or 420 nm longpass filter for Cerulean, or a 489 nm 100 mW diode laser with a 520–555 nm bandpass filter for Venus and 495–555 and 520–555 nm bandpass filter for GFP or 561 nm diode laser with a 565 nm longpass filter for mCherry. Image analysis and composite figures were prepared using ImageJ (National Institutes of Health; Bethesda, MD), Photoshop CS4 and Illustrator CS4 software (Adobe Systems, San Jose, CA). Live cell images were acquired using an Axiovert-200 wide-field fluorescence microscope (Carl Zeiss Microimaging Inc.) with a × 63/1.4 NA oil immersion objective lens, a Retiga-2000 camera (QImaging, Surrey, BC Canada), and 470/40 nm excitation, 525/50 nm emission bandpass filter for Alexa Fluor 488, 565/30 nm excitation, or 365 nm excitation, 445/50 nm emission bandpass filter for BFP. Images were acquired with QCapture software. Immunoblots and co-immunoprecipitation Total cell lysates for immunoblotting were prepared in 1% SDS, 0.1 M Tris, pH 8.0 with 100 mM DTT (reducing conditions) or no DTT (nonreducing conditions) using cells in 24-well plates at 80–90% confluence. For the reducing and nonreducing immunoblots, cells were first treated with 20 mM NEM in phosphate-buffered saline (PBS) for 15 min at room temperature. Proteins were separated using either 6 or 12% Tris-tricine gels, transferred to nitrocellulose, probed with the indicated antibodies, developed using enhanced chemiluminescent reagents (Pierce, Rockford, IL) and exposed to X-ray film. Antibodies used included anti-GFP (generous gift from Ramanujan S. Hegde, Laboratory of Molecular Biology, Cambridge, UK), anti-GAPDH (catalogue number SC25778, 1:5,000 Santa Cruz Biotechnology, Dallas, TX) and horseradish peroxidase-labelled anti-rabbit secondary antibodies (Jackson Immunoresearch Laboratories, West Grove, PA). For co-immunoprecipitation analyses, cells were cultured in six-well plates, were washed twice with PBS and lysed with Triton lysing buffer (1% Triton X-100, 50 mM HEPES, pH 7.4, 100 mM NaCl). Lysis buffers contained EDTA-free protease inhibitor cocktail (Roche, Indianapolis, IN). Lysates were clarified for 10 min at maximum speed in a microcentrifuge at 4 °C and incubated for at least 2 h at 4 °C with protein A agarose beads (Bio-Rad Laboratories, Hercules, CA) plus the indicated primary antibody. Beads were washed four times in IP lysing buffer and once in dH 2 O, eluted in SDS–polyacrylamide gel electrophoresis sample buffer and analysed on 6% SDS tricine gels, followed by immunoblot. Immunofluorescence Cells were fixed with freshly diluted 3.7% formaldehyde in PBS at room temperature for 15 min and permeabilized with 0.1% Triton X-100 in PBS. Blocking was performed with 10% fetal bovine serum in PBS for 30 min. Subsequently, cells were labelled with anti-GFP, anti-GM130 (BD Transduction Laboratories catalogue number 610823, 1:500 BD Biosciences, San Jose, CA), anti-β COP [56] (Affinity Bioreagents catalogue number PA1061, 1:500) or anti-LAMP1 (catalogue number H4A3-c 1:500, DSHB) [57] followed by Alexa Fluor 488 or 555 (as appropriate) conjugated anti-rabbit IgG secondary antibody (catalogue numbers A11008 and A21428, respectively, both used at 1:500, Life Technologies). Relative and mean fluorescence intensity quantification The relative fluorescence intensity of ER–EBFP2 and ER–oxBFP ( Fig. 3 ) was measured in transiently expressing U-2 OS cells. Images were acquired using identical imaging parameters. At least five fields of view were captured for each condition on three separate days. Images were analysed with ImageJ software. To measure a cell MFI, first the cell nucleus was excluded and detectable fluorescence signal was selected using ImageJ threshold. The average MFI values were plotted using GraphPad Prism software. To measure and compare GalT–FP levels accumulated in the ER ( Fig. 6 ), cells were fixed and stained, as above with anti-GFP followed by Alexa Fluor 555 conjugated anti-rabbit IgG secondary antibody. Images of the anti-Alexa Fluor 555 distributions were captured using identical imaging conditions and then analysed using ImageJ. Regions (10 × 10 pixels) near the GC were measured for MFI and then values were plotted using GraphPad Prism software. Protein characterization Absorbance was measured using a Hitachi U-3010 spectrophotometer (Hitachi High Technologies, Schaumburg, IL). Excitation and emission spectra were measured with a FluoroMax-3 spectrofluorometer (Horiba/Jobin Yvon, Edison, NJ). Purified protein samples were measured in PBS at room temperature. To determine extinction coefficients and quantum yields, absorbance and fluorescence of the new fluorescent variants were compared with that of parental proteins. To assess photobleaching sensitivity under comparable imaging parameters, oxFPs and parental FPs were transiently expressed in U-2 OS cells. Cells were imaged using standard live cell imaging conditions. Images were acquired at five frames per second for 400 frames. Statistical analysis Prism software (GraphPad Software, San Jose, CA) was used to compare the different conditions using two-tailed Student’s t -tests. For higher stringency, differences were not considered significant for P values >0.01. How to cite this article: Costantini, L. M. et al. A palette of fluorescent proteins optimized for diverse cellular environments. Nat. Commun. 6:7670 doi: 10.1038/ncomms8670 (2015).